Cyclic hardening in bundled actin networks Nonlinear deformations can irreversibly alter the mechanical properties of materials. Most soft materials, such as rubber and living tissues, display pronounced softening when cyclically deformed. Here we show that, in contrast, reconstituted networks of crosslinked, bundled actin filaments harden when subject to cyclical shear. As a consequence, they exhibit a mechano-memory where a significant stress barrier is generated at the maximum of the cyclic shear strain. This unique response is crucially determined by the network architecture: at lower crosslinker concentrations networks do not harden, but soften showing the classic Mullins effect known from rubber-like materials. By simultaneously performing macrorheology and confocal microscopy, we show that cyclic shearing results in structural reorganization of the network constituents such that the maximum applied strain is encoded into the network architecture. A broad range of materials exhibit dramatic and irreversible changes to their mechanical properties when deformations are large enough to elicit a nonlinear response. In many technological applications nonlinear deformations lead to undesirable changes to the material properties. In some instances, irreversible nonlinear deformations provide a simple route to in situ alterations of the material properties; as is seen in metals [1] , [2] and polymers [3] . As first reported by Mullins et al . in rubber-like materials [4] , a cyclically applied load can result in an overall softening of the material. Specifically, a lower stress is reached at strains that are lower than the maximum previously applied strain γ 0 . The softening is directly dependent on the number of cycles with the most pronounced effect occurring in the first cycle. However, if the system is sheared to a maximum strain >γ 0 , the stress-strain relation exhibits no memory of the previously applied strain. This type of softening behavior, referred to as the Mullins effect, is observed in pure and filled gums and thermoplastic elastomers [5] , as well as polymer gels [6] , living tissues [7] , [8] and biopolymer networks [9] . The microscopic origin of the Mullins effect remains unclear [5] in spite of the variety of existing models [10] . Reconstituted actin networks are ideal candidates for investigating the effect of cyclic loads at the microscopic scale using confocal fluorescence microscopy due to their large mesh sizes, and their propensity to form large bundles [11] , [12] . Interestingly, bundled actin networks also exhibit strain stiffening [11] , [13] one hallmark of materials which show the Mullins effect. From a biological perspective, insight into the response of in vitro biopolymer networks to cyclic loads may be important, as a passive reorganization induced by external mechanical stimuli should prove to be a powerful tool to facilitate the high adaptability of living materials. Here we show that the mechanical response of actin networks bundled by α-actinin or filamin in the irreversible non-linear regime exhibits strong similarities to the Mullins effect. Depending on the concentration of proteins, we not only observe Mullins-like softening, but also cyclic hardening, indicated by an irreversible increase in the nonlinear elasticity as a consequence of repeated loading cycles. Therefore, these networks show a mechano-memory—the maximal applied strain is stored in the network architecture. We simultaneously use bulk-rheology and confocal microscopy to reveal the microscopic origin of the Mullins effect and cyclic work hardening. We find that cyclic shearing causes drastic network reorganizations, such as bundling and unbundling of the fibers that is accompanied by the appearance of a negative prestrain. Cyclic hardening in actin networks bundled by α-actinin Actin networks bundled by α-actinin (actin/α-actinin networks) show a pronounced nonlinear mechanical response to external shear strains. The dependence of the differential modulus on strain in the nonlinear regime can be determined by applying a constant shear rate to the network. Above a certain strain, which is dependent on network parameters as well as external parameters like the shear rate, the network strain hardens ( Fig. 1 ); increasingly higher applied stresses are required to increase the strain. 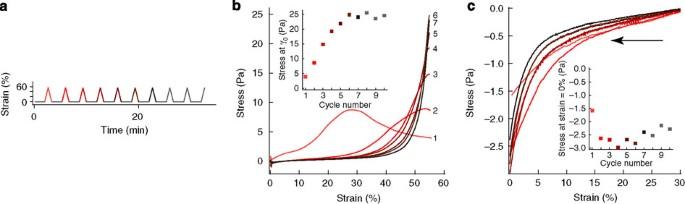Figure 1: Actin/α-actinin networks show cyclic hardening. (a) The protocol shows the cyclic shearing procedure applied to actin/α-actinin networks atca=4.75 μM,R=1 at 18 °C. The response is shown in (b,c). The networks are sheared with 1.4%/s. The responses to upward (b) and downward shearing (zoom-in shown inc) are shown for the first seven cycles in the color denoted in (a), respectively. The arrow in (c) denotes the direction of shear. The stress σ0which is reached at the maximal cyclically applied strain γ0increases as a function of cycle number (shown in the inset of (b)). The negative stress which is necessary to shear the network back to its initial position saturates after the second cycle and slightly decreases afterwards (shown in the inset of (c)). For the network with an actin concentration c a =4.75 μM and a molar ratio of cross-linking molecules to actin, R =1, at 18 °C shown in Figure 1 , we apply a continuous shear strain γ at a rate of γ ≈1.4% s −1 , the strain hardening response begins at γ ≈10% and the network withstands a maximal stress of σ max ∼ 10 Pa at γ ≈25–30%, after which a decrease of the stress is observed. Repeating the deformation a second time (according to the protocol shown in Fig. 1a ) results in a significantly different response of the network; the linear stiffness—given by the slope in the stress strain relation—decreases from ∼ 12 Pa to less than ∼ 14 Pa, the strain stiffening response starts not below γ ≈20% and a significantly sharper increase of the modulus in the nonlinear regime is observed ( Fig. 1b ). Each repetition of this deformation protocol results in an increasingly larger linear regime, a continuous decrease of the linear stiffness to ∼ 12 Pa, an increasingly larger differential modulus in the nonlinear regime and higher maximal stresses at the strain amplitude γ 0 ( Fig. 1b and inset). Thus the cyclic mechanical loading results in networks that can withstand much higher stresses. A result that is in sharp contrast to the Mullins effect which is accompanied by softening in rubber-like materials. Figure 1: Actin/α-actinin networks show cyclic hardening. ( a ) The protocol shows the cyclic shearing procedure applied to actin/α-actinin networks at c a =4.75 μM, R =1 at 18 °C. The response is shown in ( b , c ). The networks are sheared with 1.4%/s. The responses to upward ( b ) and downward shearing (zoom-in shown in c ) are shown for the first seven cycles in the color denoted in ( a ), respectively. The arrow in ( c ) denotes the direction of shear. The stress σ 0 which is reached at the maximal cyclically applied strain γ 0 increases as a function of cycle number (shown in the inset of ( b )). The negative stress which is necessary to shear the network back to its initial position saturates after the second cycle and slightly decreases afterwards (shown in the inset of ( c )). Full size image Memory effect in actin networks bundled by α-actinin Interestingly, the actin/α-actinin networks exhibit history dependence demonstrated by shearing to strains higher than γ 1 >γ 0 after such a cyclic hardening procedure ( Fig. 2 ). We observe a sharp peak in the stress-strain relation when γ is slightly above the previously applied maximum strain γ 0 . By performing additional cycles up to the new maximal strain γ 1 , the network is further cyclically work hardened; concomitantly the previous stress barrier at γ 0 is erased. As shown in Figure 3 , the cyclic hardening behavior is qualitatively independent of the strain amplitudes—as long as they are far in the non-linear regime and a significant part of the network is still connected to the surface. 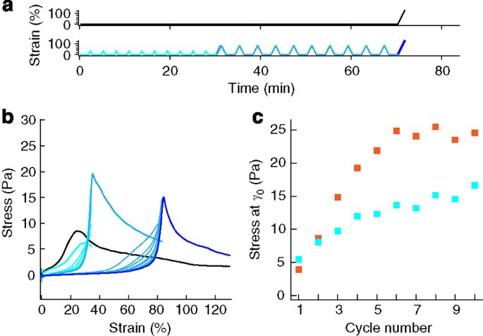Figure 3: Cyclic hardening at different strain amplitudes. The protocol and stress as a function of strain for an experiment analogous to the experiment shown inFigure 2a,bandFigure 1with different strain amplitudes is shown in (a,b). The control experiment is shown in black. Again, cyclic hardening is observed: In (c) the stress atγ0=35% as a function of cycle number (blue) is compared to cyclic hardening atγ0=56% (red) as shown in the inset ofFigure 1b. However, the saturation value of the stress at γ 0 depends on γ 0 ( Fig. 3c ). 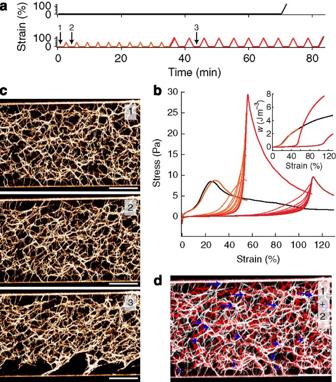The fact that the strain memory is located at the previous maximum strain and not at the maximum stress indicates that the deformation history is coded into a geometrical rearrangement of the network architecture. Figure 2: Strain induced network reorganizations explain cyclic hardening in actin/α-actinin networks. The cyclic shearing procedure applied to an actin/α-actinin network atca=4.75 μM, molar ratioR=1 at 18 °C as shown inFigure 1is extended by additional cycles at a higher amplitude and a final shearing to a third amplitude. Each color corresponds to a certain strain amplitude. Thick lines mark the first upward shearing to the respective maximum strain. (a) The complete cyclic shearing procedure as well as the control protocol (black) corresponding to the experiments shown in (b) are shown. The networks are sheared with 1.4%/s. Confocal z-stacks are taken in between the cycles, where the strain is fixed to 0%. (b) Only the response to upward shearing is shown. Inset: The total energy density necessary to shear the network up to a certain strain is shown as a function of strain. Only the first cycles to a certain strain are shown for simplicity. (c) Confocal images (x-projections of 15 μm are shown for the time points indicated in (a). (d) From the overlay image of the pictures at time point 1 (red) and time point 2 (white) it can be seen that cyclic shearing causes a negative prestrain of the network. Arrows indicate the displacement of prominent structures to the right. The network has been sheared to the left side. Shearing to the higher strain obviously causes the formation of thicker bundles (3) in (c). Scale bars denote 50 μm. A video showing one image per cycle can be seen in theSupplementary information(Supplementary Movie S1). Figure 2: Strain induced network reorganizations explain cyclic hardening in actin/α-actinin networks. The cyclic shearing procedure applied to an actin/α-actinin network at c a =4.75 μM, molar ratio R =1 at 18 °C as shown in Figure 1 is extended by additional cycles at a higher amplitude and a final shearing to a third amplitude. Each color corresponds to a certain strain amplitude. Thick lines mark the first upward shearing to the respective maximum strain. ( a ) The complete cyclic shearing procedure as well as the control protocol (black) corresponding to the experiments shown in ( b ) are shown. The networks are sheared with 1.4%/s. Confocal z-stacks are taken in between the cycles, where the strain is fixed to 0%. ( b ) Only the response to upward shearing is shown. Inset: The total energy density necessary to shear the network up to a certain strain is shown as a function of strain. Only the first cycles to a certain strain are shown for simplicity. ( c ) Confocal images (x-projections of 15 μm are shown for the time points indicated in ( a ). ( d ) From the overlay image of the pictures at time point 1 (red) and time point 2 (white) it can be seen that cyclic shearing causes a negative prestrain of the network. Arrows indicate the displacement of prominent structures to the right. The network has been sheared to the left side. Shearing to the higher strain obviously causes the formation of thicker bundles (3) in ( c ). Scale bars denote 50 μm. A video showing one image per cycle can be seen in the Supplementary information ( Supplementary Movie S1 ). Full size image Figure 3: Cyclic hardening at different strain amplitudes. The protocol and stress as a function of strain for an experiment analogous to the experiment shown in Figure 2a,b and Figure 1 with different strain amplitudes is shown in ( a , b ). The control experiment is shown in black. Again, cyclic hardening is observed: In ( c ) the stress at γ 0 =35% as a function of cycle number (blue) is compared to cyclic hardening at γ 0 =56% (red) as shown in the inset of Figure 1b . Full size image Structural reorganizations account for cyclic hardening To test this, a simultaneous observation of the structure and the mechanical response is required as a way to pinpoint the microscopic origins of the cyclic hardening behavior. Using our confocal-rheometer we provide three dimensional structural information while simultaneously measuring the mechanical response to applied shear strains. We first apply a cyclic deformation protocol to the network while acquiring confocal z-stacks after each cycle at strain γ =0 (see Fig. 2c ). Initially, the bundled network shown in Figure 2 appears homogeneous with a mesh size of ξ ∼ 12.5 μm and clearly visible attachment points of the bundles to the glass substrate with a density of ρ ∼ 5,000 mm −2 . We observe a clear structural reorganization of the network after the first deformation cycle. Indeed, the upper surface has been sheared to the left side and the attachment points of the network at the upper surface are shifted to the right side ( Fig. 2c , Supplementary Movie S1 ). The entire network structure appears as though a negative strain of roughly γ ≈−15% was applied ( Fig. 2d ). This observation is verified by the rheology. By focusing on low strains, we reveal that negative stresses of up to σ ∼ 3 Pa are required to drive the system back to its initial γ =0 position ( Fig. 1c ). In subsequent shear cycles, the network orientation no longer opposes the applied deformations. Most fibers become reorganized into structures that correspond to the spanning distance set by the previously applied strain amplitude. Therefore, the network only bears significant forces when the fibers are strongly stretched. During the subsequent cycles up to γ 0 the shear induced network reorganization becomes increasingly diminished consistent with the observation that the maximal stress reached at γ 0 is saturating with increasing cycle number ( Fig. 1b , inset) and that the necessary negative strain is saturating and decreasing with cycle number ( Fig. 1c , inset). The reorganization described above, taken together with the resulting negative prestrain, provides insights into the physical mechanism of the extended linear regime with lower stresses and the sharp increase of the modulus near γ 0 . In addition, increasingly higher stresses σ max at γ 0 are obtained and the total energy necessary to deform the network up to its complete failure is increased after the cyclic hardening procedure is performed ( Fig. 2b , inset). Due to the viscoelastic character of the network, the reorganization of attachment points could account for this effect. However, it might also indicate that a wholesale reorganization of the network constituents occurs; this is directly observed in cycles with strains to γ =112%. We observe that the cyclic shearing results in drastic bundle fusion and reorganizations while attachment points to the surface are lost thus lowering the density of attachment sites from ρ ∼ 5,000 mm −2 to only ρ ∼ 500 mm −2 . Stepwise shearing of actin networks bundled by α-actinin To better understand the process of network reorganization we apply a stepwise shear while visualizing the network response ( Fig. 4 , Supplementary Fig. S1 and Supplementary Movie S2 ). Stepwise shearing to γ 0 =56% results in continuous rupture of attachment points and an overall contraction of the network with increasing strain. The detachment from the glass appears to be cooperative; on a length scale on the order of the field of view, bonds break only at one surface while all bonds on the opposing surface remain unaffected. The observed network contraction correlates with a decrease in the measured stress ( Fig. 4c ). Shearing back to γ =0 results only in a partial relaxation of the network contraction ( Fig. 4 ). Some of the detached bundles find new contact points at the glass surface in locations where rupturing occurred. After establishing a new connection, a negative prestrain returns when the strain direction is reversed. In the subsequent deformation cycle, very few dramatic reorganization events occur. The reestablished attachment points remain in place and the network volume is almost constant and only excess lengths are extended when γ 0 =56%. Above γ 0 , rupturing, shrinkage, and reorganizations of the network are once again observed. This time most rupture events occur at the opposite—in this case the upper surface; suggesting that the reformed attachment sites at the lower surface are strengthened during the first cycle and demonstrating the cooperative nature of detachment. 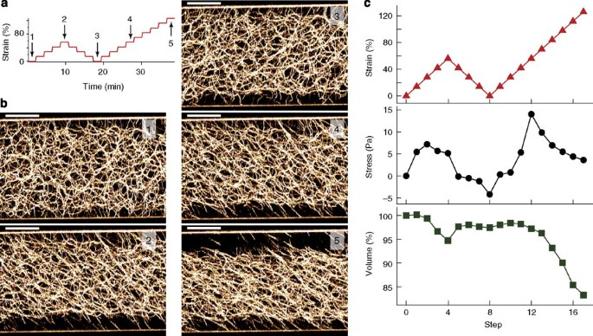Figure 4: Stepwise shearing of actin/α-actinin networks. Shearing an actin/α-actinin network atca=4.75 μM, molar ratioR=1 at 18 °C stepwise allows to image the network with a confocal microscope during cyclic loading. Indeed cyclic hardening can be observed if the network is sheared up to 56% then back to 0% and then up to a higher strain (Supplementary Fig. S1). In between the steps of 14% the strain is hold fixed for 2 min and a confocal z-stack is taken. The time points where the micrographs 1–5 have been taken are indicated in the protocol (a). (b) During the shearing of the network to 56% many bundles lose contact to the lower surface (confocal images at time points 1 and 2). An irreversible reorganization is observed when the network is sheared back (3). If the network is sheared up again, distinctly higher stresses are reached. Shearing to a higher strain results in a peak in the stress-strain relation roughly at the previous maximum strain 56%. Interestingly the network now looses contact mainly from the upper surface (5). Confocal images are x-projections of 35 μm. Scale bars denote 50 μm. A video showing one image per step can be seen in theSupplementary information(Supplementary Movie S2). (c) Strain, stress and the network volume normalized on the initial value are shown as a function of step number. As the network shrinks only in z-direction, the volume is proportional to the thickness of the network. The thickness is obtained from an intensity line profile along the z-direction and averaged over ≈250 μm in x and y direction, respectively. The position where the fluorescence intensity reaches half of the maximum value is defined as the boundary of the network. Figure 4: Stepwise shearing of actin/α-actinin networks. Shearing an actin/α-actinin network at c a =4.75 μM, molar ratio R =1 at 18 °C stepwise allows to image the network with a confocal microscope during cyclic loading. Indeed cyclic hardening can be observed if the network is sheared up to 56% then back to 0% and then up to a higher strain ( Supplementary Fig. S1 ). In between the steps of 14% the strain is hold fixed for 2 min and a confocal z-stack is taken. The time points where the micrographs 1–5 have been taken are indicated in the protocol ( a ). ( b ) During the shearing of the network to 56% many bundles lose contact to the lower surface (confocal images at time points 1 and 2). An irreversible reorganization is observed when the network is sheared back (3). If the network is sheared up again, distinctly higher stresses are reached. Shearing to a higher strain results in a peak in the stress-strain relation roughly at the previous maximum strain 56%. Interestingly the network now looses contact mainly from the upper surface (5). Confocal images are x-projections of 35 μm. Scale bars denote 50 μm. A video showing one image per step can be seen in the Supplementary information ( Supplementary Movie S2 ). ( c ) Strain, stress and the network volume normalized on the initial value are shown as a function of step number. As the network shrinks only in z-direction, the volume is proportional to the thickness of the network. The thickness is obtained from an intensity line profile along the z-direction and averaged over ≈250 μm in x and y direction, respectively. The position where the fluorescence intensity reaches half of the maximum value is defined as the boundary of the network. Full size image Cyclic hardening is sensitive to network architecture To confirm that the network reorganizations we observe are a necessary precondition for the measured strain hardening effect, we test a system with comparable microstructure that lacks the cyclic hardening response ( Fig. 5 ). 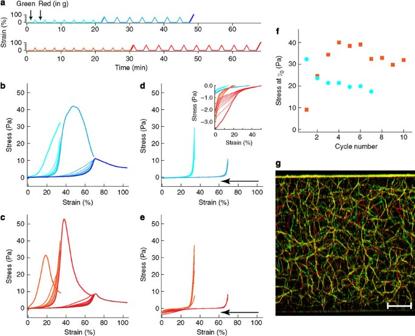Figure 5: Cyclic hardening in actin/α-actinin networks depends on protein concentrations. The cyclic hardening behavior is very sensitive to protein concentrations. Actin/α-actinin networks atca=9.5 μM,R=1 at 18 °C show a clear cyclic hardening (red—different strain amplitudes are indicated by different red colors) while it is hardly observable for actin/α-actinin networks atca=9.5 μM,R=0.5 at 21 °C (blue—different strain amplitudes are indicated by different blue colors). Thick lines mark the first upward shearing to the respective maximum strain. The responses corresponding to the protocols shown in (a) to upward and downward shearing (indicated by an arrow) are shown in (b,c) and (d,e; the inset indshows a zoom in at low strains), respectively. A shear rate of 1.4%/s and pauses of 120 s are used for both experiments. It can be seen ind,ethat for the network showing the strong cyclic hardening, distinctly higher negative stresses are reached during the downward shearing. (f) The stress at the lower cyclically applied strain 35% as a function of cycle number is shown for both networks. (g) Forca=9.5 μM,R=0.5 at 21 °C no negative prestrain results if the network is cyclically sheared to 35%/s. The micrograph shows an overlay of confocal images (x projections 21 μm before (green) and after (red) the first cycle as indicated in a)). Scale bar denotes 25 μm. The protocol observed is described in Figure 5a , whereas the responses to strain are depicted in Figure 5b–e . Networks with a lower effective α-actinin concentration exhibit a cyclic softening in accordance with the classic Mullins effect ( Fig. 5b,f ) and do not show dramatic reorganizations with an encoding of a prestrain ( Fig. 5g ). However, through the cyclic shearing process, some attachments to the surface are lost, which may explain the observed similarity to the Mullins effect. The stress necessary to shear the network back to its initial position is compared with that of a network with an effectively higher α-actinin concentration, which shows the cyclic hardening effect. For the network that hardens, the negative stresses reached at γ =0 are far higher than for the network with the lower α-actinin concentration ( Fig. 5d,e )—although the maximum positive stresses which are reached during the cyclic shearing procedure are comparable in magnitude for both networks ( Fig. 5b,c ). This supports that the negative prestrain observed with confocal microscopy accounts for the negative stresses and contributes to the cyclic hardening effect. Figure 5: Cyclic hardening in actin/α-actinin networks depends on protein concentrations. The cyclic hardening behavior is very sensitive to protein concentrations. Actin/α-actinin networks at c a =9.5 μM, R =1 at 18 °C show a clear cyclic hardening (red—different strain amplitudes are indicated by different red colors) while it is hardly observable for actin/α-actinin networks at c a =9.5 μM, R =0.5 at 21 °C (blue—different strain amplitudes are indicated by different blue colors). Thick lines mark the first upward shearing to the respective maximum strain. The responses corresponding to the protocols shown in ( a ) to upward and downward shearing (indicated by an arrow) are shown in ( b , c ) and ( d , e ; the inset in d shows a zoom in at low strains), respectively. A shear rate of 1.4%/s and pauses of 120 s are used for both experiments. It can be seen in d , e that for the network showing the strong cyclic hardening, distinctly higher negative stresses are reached during the downward shearing. ( f ) The stress at the lower cyclically applied strain 35% as a function of cycle number is shown for both networks. ( g ) For c a =9.5 μM, R =0.5 at 21 °C no negative prestrain results if the network is cyclically sheared to 35%/s. The micrograph shows an overlay of confocal images (x projections 21 μm before (green) and after (red) the first cycle as indicated in a)). Scale bar denotes 25 μm. Full size image Cyclic hardening in actin networks bundled by filamin To test if the high binding propensity of α-actinin is a precondition for the observed reorganization and cyclic hardening behavior [12] , [14] , we also utilize the actin crosslinking protein filamin, a protein that kinetically traps actin networks similar to α-actinin [15] . The architecture of the bundled actin/filamin networks, at the concentrations chosen, resembles that of actin/α-actinin networks. Interestingly, cyclic shearing of actin/filamin networks also results in hardening ( Fig. 6 ). In contrast to the response of actin/α-actinin networks the stress reached at the maximal cyclically applied strain γ 0 decreases as a function of the cycle number ( Fig. 6c )—in accordance with the classic Mullins effect. However, if the network is sheared to larger strains significantly higher stresses than in the control measurement are obtained. Also, stepwise shearing of the network results in a higher maximum stress if a single stepwise cycle to a lower strain is previously applied ( Supplementary Fig. S2 ). Confocal imaging reveals that cyclic shearing not only results in a negative prestrain, but in addition the actin/filamin bundles are partially unbundled. 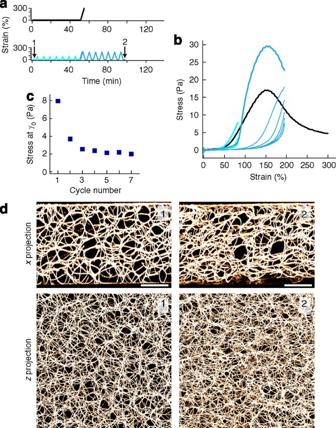Figure 6: Cyclic hardening in actin/filamin networks. Actin/filamin networks atca=9.5 μM,R=0.1 at 21 °C show cyclic hardening. (a) The protocol for the control experiment (black) and the cyclic shearing procedure (blue—different strain amplitudes are indicated by different blue colors) are shown. Thick lines mark the first upward shearing to the respective maximum strain. (b) The black line shows the network response to a constant shear rate 1.4%/s. Blue colors show the response to the cyclic shearing procedure shown in (a). Thick lines show the response to the first cycle applied up to the respective maximum strain. Only the response to upward shearing is shown. At the maximal cyclically applied strain the stress decreases as a function of cycle number (c). Higher stresses are reached beyond this strain (b). (d) Confocal images (x projection of 63 μm; z projection of 130 μm—surface near regions are not shown in order to reduce the background fluorescence) which are taken during the experiment (time points where the images are taken are indicated in the protocol (a)) reveal that cyclic shearing causes unbundling. A larger number of thin bundles appears and the mesh size decreases. Scale bars denote 50 μm and are also valid for z-projections. Videos showing one image per cycle can be seen in theSupplementary Movie S3andS4. As shown in Figure 6d and Supplementary Movie S3 and S4 , a larger number of thin bundles is observed after the cyclic shearing procedure resulting in a decrease in the mesh size. Quantitative image analysis reveals that the mesh size of the network shown in Figure 6 decreases from initially 34.3 to 27.4 μm at time point 2 (see Fig. 6 ). One potential consequence of the unbundling is an increase in the length of bundle-paths percolating between the surfaces. Thus, the cyclic training results in bundles which are longer than the maximal cyclically applied strain would imply. In this scenario, higher strains have to be applied to fully stretch bundles and detach them from the surface. This causes that the sharp increase of stress is seen at higher strains, while the stress reached at γ 0 decreases. Figure 6: Cyclic hardening in actin/filamin networks. Actin/filamin networks at c a =9.5 μM, R =0.1 at 21 °C show cyclic hardening. ( a ) The protocol for the control experiment (black) and the cyclic shearing procedure (blue—different strain amplitudes are indicated by different blue colors) are shown. Thick lines mark the first upward shearing to the respective maximum strain. ( b ) The black line shows the network response to a constant shear rate 1.4%/s. Blue colors show the response to the cyclic shearing procedure shown in ( a ). Thick lines show the response to the first cycle applied up to the respective maximum strain. Only the response to upward shearing is shown. At the maximal cyclically applied strain the stress decreases as a function of cycle number ( c ). Higher stresses are reached beyond this strain ( b ). ( d ) Confocal images (x projection of 63 μm; z projection of 130 μm—surface near regions are not shown in order to reduce the background fluorescence) which are taken during the experiment (time points where the images are taken are indicated in the protocol ( a )) reveal that cyclic shearing causes unbundling. A larger number of thin bundles appears and the mesh size decreases. Scale bars denote 50 μm and are also valid for z-projections. Videos showing one image per cycle can be seen in the Supplementary Movie S3 and S4 . Full size image The fact that also for actin/filamin bundle networks cyclic loads result in irreversible structural reorganizations which manifest themselves in the non-linear mechanical response, suggests that this might be a typical feature of kinetically trapped actin bundle networks. Using confocal-rheology, we reveal that bundled actin networks demonstrate a significant mechanical history dependence, which is encoded into the network architecture as a strain memory. This sets the mechanical response of these biopolymer networks. At low concentrations of the crosslinking protein α-actinin, a cyclic softening is observed, similar to the classic Mullins [5] . By simultaneously recording the rheology while visualizing the mechanical response of bundled actin networks, the classic Mullins effect is traced back to detachments of bundles. In contrast, strongly crosslinked α-actinin networks show a pronounced cyclic hardening behavior. Cyclic shearing results in a reorganization of the network architecture accompanied by the development of a negative prestrain and a reorganization of the network constituents. Shearing enables a reorganization of the bundles through a disruption of network structures that leads to new contacts being formed between bundles. The surface-network interface seems to play an important role for the shear induced network reorganization. The most drastic rupture events occur at the surface—this is presumably the case because these links are the weakest in the system. A remaining challenge is understanding the intricate balance between rupturing events, reorganization and prestrain and their combined consequence for the mechanical response. The high binding propensity of the α-actinin and filamin coupled with their tendency to kinetically trap actin networks seem to be a prerequisite for the observed effects; actin networks cross-linked by other cross-linking proteins, such as fascin or HMM do not cyclically harden at the conditions we tested. Cyclic work hardening is not expected for flexible polymers [16] . However, we show that semi-flexible polymers bundled by transient cross-links demonstrate work hardening and mechano-memory. Such a smart material may be interesting for the ability to adapt to repeated deformations. Our experiments demonstrate that rather simple composite biological systems consisting of solely actin and cross-linking proteins passively adapt their structural and mechanical properties upon external mechanical stimuli. Living cells may make use of such mechanisms to adapt or reorganize cytoskeletal structures through external mechanical stimuli. We speculate that a strain memory effect, where the material drastically softens within an applied strain range, but exhibits a high stress barrier at higher strains, might be utilized in biological systems to allow for movement in a certain but adaptable range while maintaining mechanical stability. Protein purification G-actin is obtained from rabbit skeletal muscle by a modified protocol of ref. 17 , where an additional gel filtration (Sephacryl S-300 HR) as well as an additional polymerization-depolymerization step is done. The actin is stored in lyophilized form at −21 °C [17] . The G-actin solution is prepared by dissolving lyophilized actin in deionized water and dialyzing against G-buffer (2 mM Tris, 0.2 mM ATP, 0.2 mM CaCl 2 , 0.2 mM DTT and 0.005% NaN 3 , pH 8) at 4 °C. The G-actin solution is kept at 4 °C and is used within two weeks. Polymerization is initiated by adding 10% volume 10x F-buffer (20 mM Tris, 5 mM ATP, 20 mM MgCl 2 , 2 mM CaCl 2 , 1 M KCl, 2 mM DTT, pH 7.5). For confocal imaging, actin is labelled with Atto 488 phalloidin (Invitrogen). α-actinin is isolated from turkey gizzard smooth muscle following [18] , dialyzed against G-buffer and stored at 4 °C for several weeks. Muscle filamin is isolated from chicken gizzard, and further purified as reported in ref. 19 . Confocal rheology Experiments are performed with a Leica TCS SP5 point-scanning confocal microscope coupled to a modified Anton Paar MCR 301 stress-controlled rheometer. A plate cone geometry is used. The metal cone is rinsed with H 2 O and wiped ten times prior to use. A fresh glass cover slip which has been rinsed with H 2 O is used as lower plate. For the cyclic hardening procedure strain is controlled. After upward and downward shearing with constant shear rate, strain is kept at 0% in the pauses between the cycles. Similarly, strain is kept constant in the pauses of stepwise shear experiments. The confocal-rheometer coupling allows us to image three-dimensional volumes of the network over time while simultaneously applying a precisely controlled shear strain. Image analysis We characterize the mesh size of the networks by quantifying the spatial separation between filaments extracted along horizontal and vertical lines within thresholded z-resolved planar confocal images. We fit the distribution of filament spacing to an exponential decay to obtain an estimate of the characteristic length scale describing the network mesh or pore size [20] . The number of attachment sites at the surface is determined by counting within a representative area. How to cite this article: Schmoller, K.M. et al . Cyclic hardening in bundled actin networks. Nat. Commun. 1:134 doi: 10.1038/ncomms1134 (2010).